Highly transparent nonvolatile resistive memory devices from silicon oxide and graphene Transparent electronic memory would be useful in integrated transparent electronics. However, achieving such transparency produces limits in material composition, and hence, hinders processing and device performance. Here we present a route to fabricate highly transparent memory using SiO x as the active material and indium tin oxide or graphene as the electrodes. The two-terminal, nonvolatile resistive memory can also be configured in crossbar arrays on glass or flexible transparent platforms. The filamentary conduction in silicon channels generated in situ in the SiO x maintains the current level as the device size decreases, underscoring their potential for high-density memory applications, and as they are two-terminal based, transitions to three-dimensional memory packages are conceivable. As glass is becoming one of the mainstays of building construction materials, and conductive displays are essential in modern handheld devices, to have increased functionality in form-fitting packages is advantageous. Potential technological advances from visibly transparent circuits have aroused extensive interest and motivated various studies [1] , [2] . Progress has been made by using wide-bandgap semiconductors or nanowires to construct transparent transistors [3] , [4] , [5] , [6] . For the realization of a fully integrated transparent circuit, high transparency is also desirable in one of the other circuitry elements: the memory unit. Although charge-based transparent memory can be constructed based on the transistor structure [7] , [8] , [9] , it comes with the tradeoff in nonvolatility due to the limitations in achieving both high transparency and efficient charge trapping in the floating gate. This sacrifice can be eliminated using resistive switching memory that functions on a non-charge-based mechanism [10] , provided that transparency is achieved both in the resistance-change (active) material and the electrodes. Although this search has recently been done in metal oxides and organic materials [11] , [12] , [13] , a high-transparency memory device based on more conventional materials is desirable for processing and application reasons. Using silicon oxide (SiO x , x ~2) and graphene, the former a ubiquitous material favoured by the semiconductor industry and the latter a promising two-dimensional conductor [14] , we demonstrate here a nonvolatile memory device featuring both high transparency and robust retention, further implemented on a flexible plastic substrate. This new set of physical parameters, transparency with flexibility, could open the door for greater functionality in form-conforming packages. For optical transparency without sacrificing the memory density or capacity, intrinsic transparency is required in the single memory unit. This requirement precludes many resistance-change materials with a bandgap <3.1 eV (ref. 1 ). For the vertical sandwiched structure adopted in resistive switching memory [10] , the transparency can be further compromised by the top and bottom electrodes. For this reason, although transparent solid electrolytes can be involved in some metallic programmable cells [10] , [15] , the need for a metal electrode as the filament-injection source limits the transparency in the device unit. Similarly, the requirement of a specific electrode–material interface in some other resistive switching systems [16] restricts the choice of transparent electrode materials. As the mechanisms in many resistive switching systems have not yet been fully understood [16] , particularly with respect to the role of the electrode, the assessment of the potential application in transparent electronics depends on the actual demonstration. As one of the backbones of the semiconductor industry, SiO x comes with the advantages in both its material composition and facile processing. With a large bandgap (~9 eV), it also features high transparency. Instead of merely serving as a passive solid electrolyte in metallic programmable cells [15] , an active role of SiO x in constructing resistive switching memory was recently revealed: SiO x itself can serve as the source of the formation of metallic-phase silicon filaments as well as the surrounding supportive matrix [17] , [18] . The result is a memory effect that is intrinsic to SiO x and largely electrode independent [19] , [20] . This intrinsic memory effect in SiO x relaxes the restriction on the choice of electrode materials, making high-transparency memory devices feasible. Graphene/SiO x /indium tin oxide (ITO) devices We first chose graphene and ITO as the top and bottom electrode materials, respectively. Graphene represents a new class of two-dimensional material that is promising for future transparent electronics [21] , whereas ITO represents the mainstream choice for transparent conductive materials. The combination of the two electrode materials in a single device demonstrates the versatility of the SiO x -based memory with respect to the choice of transparent electrode materials. Vertical sandwiched pillar structures of G/SiO x /ITO (here G denotes graphene) were defined on a glass substrate ( Fig. 1a ). Specifically, the SiO x layer (~70 nm thick) was prepared by physical vapour deposition on a glass substrate coated with a layer of ITO (~120 nm thick), with the top electrode consisting of bilayer graphene prepared by the chemical vapour deposition method and transfer process [22] . Photolithography and reactive ion etching were then used to define the circular G/SiO x /ITO memory units at a diameter of ~100 μm for an easy probe-tip landing ( Supplementary Fig. S1 ). The electrical characterizations were performed in vacuum (10 −5 Torr) at room temperature in a probe station connected to an Agilent 4155C semiconductor parameter analyser. 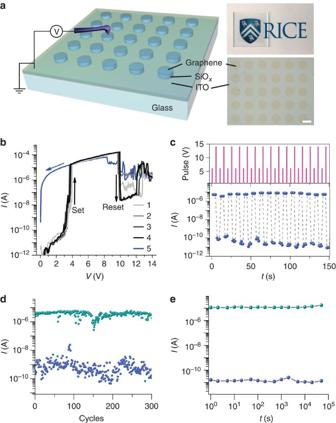Figure 1: Memory effect in a G/SiOx/ITO device. (a) Left panel: schematic of the G/SiOx/ITO device arrays on a glass substrate and the setup for electrical characterization. The top right panel shows the G/SiOx/ITO-layered structure on a glass substrate and the bottom right panel shows the optical images of the G/SiOx/ITO devices; scale bar, 100 μm. (b)I–Vcurves from an electroformed G/SiOx/ITO device, with the numbers indicating the voltage-sweep orders. Curves 1–4 are forward voltage sweeps (0→14 V), and curve 5 is backward voltage sweep (14→0 V). The voltage sweep rate is 2.8 V s−1for this and the otherI–Vcurves in this paper. (c) (Top panel) A series of voltage pulses of +6 V, +1 V (five times) and +14 V serve as set, read (five times) and reset operations, respectively. (Bottom panel) Currents corresponding to each read pulse in the top panel. (d) 300 memory cycles in a G/SiOx/ITO device. (e) Retention of the memory state tested by continuous +1 V voltage pulses (at a rate of 1 pulse per second) for both an ON and an OFF state. Figure 1: Memory effect in a G/SiO x /ITO device. ( a ) Left panel: schematic of the G/SiO x /ITO device arrays on a glass substrate and the setup for electrical characterization. The top right panel shows the G/SiO x /ITO-layered structure on a glass substrate and the bottom right panel shows the optical images of the G/SiO x /ITO devices; scale bar, 100 μm. ( b ) I–V curves from an electroformed G/SiO x /ITO device, with the numbers indicating the voltage-sweep orders. Curves 1–4 are forward voltage sweeps (0→14 V), and curve 5 is backward voltage sweep (14→0 V). The voltage sweep rate is 2.8 V s −1 for this and the other I–V curves in this paper. ( c ) (Top panel) A series of voltage pulses of +6 V, +1 V (five times) and +14 V serve as set, read (five times) and reset operations, respectively. (Bottom panel) Currents corresponding to each read pulse in the top panel. ( d ) 300 memory cycles in a G/SiO x /ITO device. ( e ) Retention of the memory state tested by continuous +1 V voltage pulses (at a rate of 1 pulse per second) for both an ON and an OFF state. Full size image Figure 1b shows a series of current–voltage ( I–V ) curves from a G/SiO x /ITO device after the electroforming process ( Supplementary Fig. S2 ). In the characteristic I–V curve (black curve), starting from a high-resistance (OFF) state, the current level suddenly increases at ~4 V to a low-resistance (ON) state and then decreases at ~10 V. The current or conductance increase and decrease define the set and reset values, respectively [17] , [20] , indicating unipolar resistive switching behaviour. The resistance or memory state can be read at a low-voltage bias (<3 V) without altering its value, featuring the nonvolatile property. Figure 1c,d shows a series of memory cycles using +1, +6 and +14 V as read, set and reset voltages, respectively. Note that more detailed mechanistic discussions with respect to the phenomenological behaviours of the set and reset processes can be found in ref. 18 . The nonvolatility or memory retention was tested by continuous memory-state readout at + 1 V, which showed no degradation after 5×10 4 s ( Fig. 1e ). This is consistent with our previous study showing that the memory state is robust in ambient environment for more than 3 months [23] . After testing more than 20 devices, a device yield of ~70% was achieved for the tested memory units, discounting the possibility of a contamination-related memory effect. The device failure is defined as either the failure to electroform the device (up to 40 V) or a state of non-switchable conducting (short circuited) after the attempt of electroforming. However, this depressed yield compared with that achieved in devices with polysilicon electrodes [17] is likely caused by the atomically thin nature of the graphene electrode, as structural damage in the graphene layer might result during the processing and/or the probe-tip landing processes, during which the contacting pressure could not be well monitored ( Fig. 1a ). The resultant damage could cause sliding of the graphene electrode towards the etched edge region of the device or the direct puncture and penetration of oxide, and hence, shorting of the devices, thereby lowering the yield. Note that the possibility of extrinsic switching through metal filament formation from the tungsten probe tip in contact with the top electrode was ruled out by control experiments in which memory switching could not be achieved in devices that were devoid of the top graphene electrodes ( Supplementary Fig. S3 ). Note that the I–V curves in the reset region generally involve current fluctuations [23] (blue curve, Fig. 1b ), which prevent a clear definition of the threshold value of the reset voltage. The current fluctuations are indications of the dynamic and competing effects between the set and reset processes [18] . We therefore performed a series of measurement on the set voltages, as well as the ON and OFF currents, showing a comparatively narrow distribution of the set voltages (4.26±0.54 V) and the ON/OFF ratios are between 10 3 and 10 6 ( Supplementary Fig. S4 ). G/SiO x /G devices The intrinsic memory switching in SiO x enables the construction of completely metal-free transparent memory devices by using graphene as the only electrode material. For the fast progress in synthesis and abundance in the carbon sources [24] , [25] , [26] , graphene has become a promising candidate for transparent electrode materials [21] , [25] . The use of graphene and SiO x , another low-cost and industry-standard material, as the only materials for constructing memory devices, therefore, comes with the advantages both in the material composition and processing. This is in contrast to other transparent resistive switching memory based on traditional metal-oxide materials [11] , [12] , [13] , for which low-cost replacements such as graphene have been sought [21] , [25] . As shown in Fig. 2a , vertical sandwiched pillar structures of G/SiO x /G with the same diameters (~100 μm) were defined on the glass substrate ( Supplementary Fig. S5 ), which shows 90% transparency at 550 nm ( Fig. 2b ). Specifically, bilayer graphene sheets were used for both the top and bottom electrodes with the SiO x thickness ~70 nm. The devices showed similar resistive switching I–V curves and memory property ( Fig. 2c,d ) to those exhibited in Fig. 1 at a yield of 65% with over 20 devices being tested; the 35% non-operating devices being short circuited. The use of graphene as both top and bottom electrodes further indicates the intrinsic memory property of SiO x by excluding the possibility of metal filament formation from the electrode materials. Note that although graphene and graphene oxide have been used in some resistive switching systems, the inevitable use of metal electrodes limits the transparency of the memory devices [27] , [28] . Because of the low optical absorbance in graphene [29] , uniform transmittance as high as ~90% over the entire visible range is achieved in the G/SiO x /G devices ( Fig. 2b ). Note that here bilayer graphene was used for both the top and bottom electrodes for the purpose of better coverage. It is not due to an intrinsic limit with respect to the resistance. In fact, as the ON-state resistance of SiO x is ≫ 10 kΩ ( Fig. 2d ), doped monolayer graphene (<1 kΩ sq −1 ) [21] can serve as the electrode material. As a result, the transmittance can be further increased to ~95% (blue curve, Fig. 2b ), which is higher and more uniform than those achieved in other systems [11] , [12] , [13] , [30] . 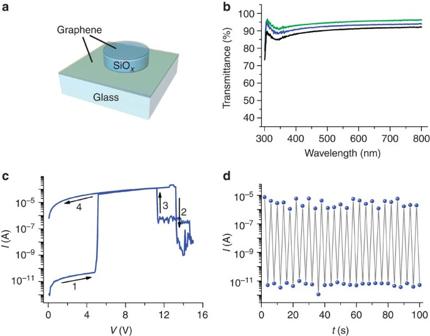Figure 2: Memory effect in a G/SiOx/G device. (a) Schematic of the G/SiOx/G device on glass. (b) Optical transmittance in G/SiOx/G-layered structures with different layer thicknesses of graphene. The green, blue and black curves correspond to the transmittance in MLG/SiOx/MLG, MLG/SiOx/BLG and BLG/SiOx/BLG structures. Here BLG and MLG denote bilayer graphene and monolayer graphene, respectively. (c) CharacteristicI–Vcurves from an electroformed G/SiOx/G device. The arrows indicate the voltage-sweep directions and the numbers indicate the order. (d) Corresponding memory cycles from the device using +6 and +15 V as set and reset voltages, respectively. The programming current is not shown here and the memory states (current) were recorded at +1 V. Figure 2: Memory effect in a G/SiO x /G device. ( a ) Schematic of the G/SiO x /G device on glass. ( b ) Optical transmittance in G/SiO x /G-layered structures with different layer thicknesses of graphene. The green, blue and black curves correspond to the transmittance in MLG/SiO x /MLG, MLG/SiO x /BLG and BLG/SiO x /BLG structures. Here BLG and MLG denote bilayer graphene and monolayer graphene, respectively. ( c ) Characteristic I–V curves from an electroformed G/SiO x /G device. The arrows indicate the voltage-sweep directions and the numbers indicate the order. ( d ) Corresponding memory cycles from the device using +6 and +15 V as set and reset voltages, respectively. The programming current is not shown here and the memory states (current) were recorded at +1 V. Full size image Although the vertical pillar structures adopted above are frequently used for single-device testing purpose [16] , the implementation of the memory device relies on the construction of crossbar arrays [10] , [16] . We further demonstrate the transparent SiO x crossbar memory arrays with graphene serving as both the electrode and interconnect material, in this case constructed atop a silicon/silicon oxide substrate. 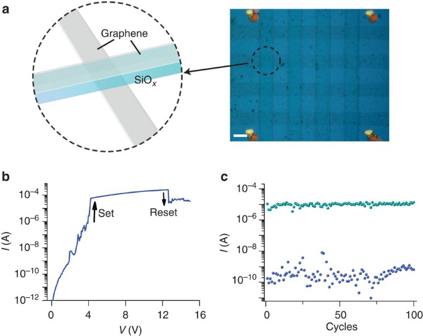Figure 3: Memory effect in a G/SiOx/G crossbar structure. (a) Optical image of the 4×4 G/SiOx/G crossbar structure (right panel), with the illustration showing the perspective view of the memory unit. Scale bar, 20 μm. (b) CharacteristicI–Vcurves from an electroformed crossbar memory unit. (c) 100 memory cycles from the device using +5 and +15 V as set and reset voltages, respectively. The programming current is not shown here and the memory states (current) were recorded at +1 V. Figure 3a shows a 4×4 SiO x crossbar structure with the SiO x (~70 nm thick) sandwiched between the top and bottom bilayer graphene lines. Figure 3b,c show the typical I–V curve and memory switching cycles from one of the crossbar units (20×20 μm 2 ), featuring the same switching characteristics as those shown in the vertical pillar structures. The observed ON and OFF currents fall into the same range as those observed in vertical pillar structures ( Supplementary Fig. S4 ). The crossbar structure with both the top and bottom electrodes extended through the graphene lines avoids the direct contact between the probe tip and the memory unit during the electrical testing, which eliminates the possibility of metal contamination from the probe tip and, hence, further confirms the intrinsic memory effects in SiO x . This may have also contributed to an increased device yield to ~80% (16 of 20 devices) due to the absence of damage from the probe tip to the graphene electrodes as discussed before. The SiO x memory here features low programming current levels (~0.1 mA, Fig. 3b ), more than one order of magnitude lower than those in other transparent resistive memory systems [11] , [12] , [13] , [30] . Consequently, despite a working voltage up to 15 V, the devices still feature an approximately tenfold reduction in the power-consumption factor (the product of current and voltage) during programming compared with those in other transparent resistive memories [11] , [12] , [13] . The reduced programming currents lower the current densities in the interconnects, providing more area for the transparent interconnects for a transparent circuit. Figure 3: Memory effect in a G/SiO x /G crossbar structure. ( a ) Optical image of the 4×4 G/SiO x /G crossbar structure (right panel), with the illustration showing the perspective view of the memory unit. Scale bar, 20 μm. ( b ) Characteristic I–V curves from an electroformed crossbar memory unit. ( c ) 100 memory cycles from the device using +5 and +15 V as set and reset voltages, respectively. The programming current is not shown here and the memory states (current) were recorded at +1 V. Full size image The versatile transfer process of graphene to various substrates [21] also enables the fabrication of the memory devices on plastic transparent films. We fabricated G/SiO x /G devices using both crossbar and pillar structures on a plastic (fluoropolymer, PFA) substrate ( Fig. 4a,b ). Here a fluoropolymer was chosen as the plastic substrate for its comparatively high-melting point (>280 °C) in order to sustain the current local heating involved during the initial electroforming process in the G/SiO x /G devices. The electroformed devices showed the same memory switching characteristics ( Fig. 4c and Supplementary Fig. S6a ) as those from devices on rigid substrates. Similar device yields of ~70% were achieved in the crossbar structures ( Fig. 4a ). The yield was comparatively low (~20%) for the pillar structures ( Fig. 4b ); the lowered yield in the pillar structure was largely due to the direct contacting between the probe tip and the memory unit during electrical characterization. Unlike the rigid substrate, the flexibility in the plastic substrate made control of the contacting pressure between the probe tip and device surface difficult, and probe-tip-induced local curvature of the device likely resulted in damage to the SiO x layer and, hence, the decreased yield. Both structures showed no memory-state degradation on bending the flexible plastic substrate ( Fig. 4d and Supplementary Fig. S6b ), demonstrating the feasibility of both transparent and flexible memory applications. 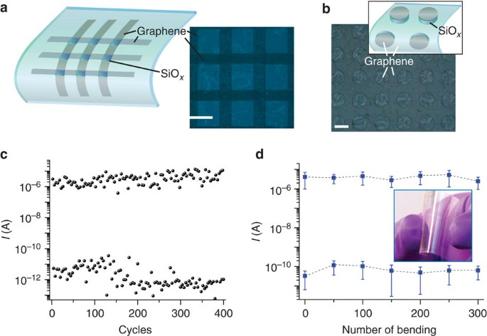Figure 4: Flexible transparent memory devices. (a) (Left panel) Schematic of the G/SiOx/G crossbar structures on a plastic (fluoropolymer) substrate and (right panel) the optical image of the structures. Scale bar, 20 μm. (b) Optical image of the G/SiOx/G pillar structures with the inset showing the schematic image. Scale bar, 100 μm. (c) Memory cycles from one of the crossbar devices using +5 and +14 V as set and reset voltages, respectively. The programming current is not shown here and the memory states (current) were recorded at +1 V. (d) Retention of both ON and OFF memory states (read at +1 V) from a crossbar device is shown on bending the plastic substrate around a ~1.2-cm diameter curvature; the central devices on the sheet being tested throughout the bending cycles. The inset shows the actual transparent memory devices using the pillar structures on the plastic substrate. Figure 4: Flexible transparent memory devices. ( a ) (Left panel) Schematic of the G/SiO x /G crossbar structures on a plastic (fluoropolymer) substrate and (right panel) the optical image of the structures. Scale bar, 20 μm. ( b ) Optical image of the G/SiO x /G pillar structures with the inset showing the schematic image. Scale bar, 100 μm. ( c ) Memory cycles from one of the crossbar devices using +5 and +14 V as set and reset voltages, respectively. The programming current is not shown here and the memory states (current) were recorded at +1 V. ( d ) Retention of both ON and OFF memory states (read at +1 V) from a crossbar device is shown on bending the plastic substrate around a ~1.2-cm diameter curvature; the central devices on the sheet being tested throughout the bending cycles. The inset shows the actual transparent memory devices using the pillar structures on the plastic substrate. Full size image Planar G–SiO x –G nanogap devices Although the transparent memory devices demonstrated above all use the common vertical sandwiched structures, they can also be made in the planar configuration. Topologically, the vertical G–SiO x –G structure is equivalent to the planar G–SiO x –G nanogap system ( Fig. 5a ). For the demonstration, we transferred graphene onto a silicon substrate capped with 500-nm-thick SiO 2 . The graphene layer was patterned with electron-beam lithography and then etched into stripes and then contacted by electrodes (2 nm Ti/30 nm Au) with a channel length ~2 μm (top panel, Fig. 5b ). Electrical breakdown was induced ( Supplementary Fig. S7a ) in the graphene stripe to generate a narrow disruption region or nanogap [19] (bottom panel, Fig. 5b ). The size of the nanogap is usually 10–60 nm, close to the thickness of SiO x layer used in the vertical G/SiO x /G devices. The electroforming of SiO x in the nanogap ( Supplementary Fig. S7b ) region usually occurs immediately after the breakdown event in the graphene stripe, most likely due to the existence of local confinement so that high field is easily attained locally. It features a reduced electroforming voltage compared with the typical value obtained from the pristine vertical structure ( Supplementary Fig. S2 ). This material-assisted local-field enhancement offers another route to bring down the electroforming voltage apart from thermal annealing [17] . As a result, a thin layer of conducting molecules or carbon materials could be coated over the SiO x surface region to induce local-field enhancement for reduction of the electroforming voltage [20] . The switching properties obtained in this planar nanogap configuration are similar to those from vertical structures, confirming the same switching mechanism intrinsic to SiO x [18] . Note that more detailed discussions about this intrinsic SiO x switching mechanism are covered in our previous studies [17] , [18] , [19] , [20] . 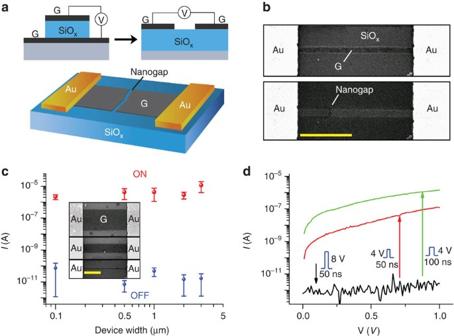Figure 5: Device scaling and switching speed. (a) Schematics of the topological equivalence between a vertical G/SiOx/G structure and a planer nanogap system. The bottom panel is a perspective view of the planar structure. (b) (Top panel) Scanning electron microscopy (SEM) image of the as-made graphene stripe device before electrical characterization. (Bottom panel) SEM image of the same device after electrical breakdown in the graphene stripe, showing a voltage-induced disruption region or nanogap; scale bar, 1 μm. (c) ON and OFF currents with respect to different lateral constrictions (widths) in the G/SiOx/G planar nanogap switching systems. The memory states were read by +1 V voltage. The inset shows a series of devices with different widths in the graphene stripes; scale bar, 1 μm. (d) Switching-speed test from one of the G/SiOx/G devices. The arrows indicate the directions of the memory-state transitions. The rising edge and falling edge of the pulses were 10 ns. Figure 5: Device scaling and switching speed. ( a ) Schematics of the topological equivalence between a vertical G/SiO x /G structure and a planer nanogap system. The bottom panel is a perspective view of the planar structure. ( b ) (Top panel) Scanning electron microscopy (SEM) image of the as-made graphene stripe device before electrical characterization. (Bottom panel) SEM image of the same device after electrical breakdown in the graphene stripe, showing a voltage-induced disruption region or nanogap; scale bar, 1 μm. ( c ) ON and OFF currents with respect to different lateral constrictions (widths) in the G/SiO x /G planar nanogap switching systems. The memory states were read by +1 V voltage. The inset shows a series of devices with different widths in the graphene stripes; scale bar, 1 μm. ( d ) Switching-speed test from one of the G/SiO x /G devices. The arrows indicate the directions of the memory-state transitions. The rising edge and falling edge of the pulses were 10 ns. Full size image This planar G-SiO x -G structure offers an easy way to study the current-scaling property by varying the widths of the graphene stripes. As shown in Fig. 5c , both the ON and OFF currents stayed at the same level when reducing the width from 3 μm to 100 nm. And these current levels are similar to those obtained in vertical structures having dimensions ≥10 μm. This non-scaling feature in the current indicates that the memory switching is through a highly localized filament. Indeed, the metallic silicon filament was revealed to be sub-10 nm in size [17] , [18] , being a possible harbinger of aggressive device scaling. This confined nanoscale switching along with the intrinsic transparency shows the possibility of high-density transparent memory applications. We further performed a switching-speed test in the G/SiO x /G devices by using a voltage–pulse generator (Agilent, B1525A). For the three G/SiO x /G devices tested, they all could be reset by a 50-ns 8 V pulse (black curve, Fig. 5d ). The set process was found to be in the range of 50–500 ns, showing variations between devices and individual switching events in the same device. The switching speed differences indicate structural and, hence, switching dynamics variations in the silicon filaments. Figure 5d shows the typical trend that a shorter (50 ns, 4 V) pulse can partially set the device (red curve), whereas a longer one (100 ns , 4 V) fully sets the device into the ON state (green curve). Note that our recent in situ imaging study [18] revealed that the switching is due to the transition between the metallic form and amorphous form in the silicon filament, with the set and reset processes largely being field driven and thermal driven, respectively. Our test indicates that the reset process (amorphization of silicon by a thermal process [18] ) is generally faster than the set process (crystallization of the silicon by a field process [18] ). This trend is analogous to that in phase-change materials, in that the set process generally requires longer programming time [31] . The partially set process (or intermediate state) by shorter pulse indicates a continuous structural evolution instead of a threshold change in the filament during the set (crystallization) process. It further bespeaks of the possibility for multi-states on a singular device. Note that Fig. 1b (blue curve) indicates that a backward voltage sweep ( V reset → 0 V) at a slow rate (~3 V s −1 ) sets the device ON, as it bypasses the set region. As the falling edge in a reset pulse is analogous to a backward sweep ( Supplementary Fig. S8 ), the fast set process observed here indicates that a fast-falling edge is necessary for the reset process ( Supplementary Discussion ). In summary, we have demonstrated transparent nonvolatile memory devices based on SiO x and graphene, which feature high transparency, long retention time and low programming currents. The underlying mechanism is a memory switching intrinsic to SiO x [17] , [18] , so that it is not limited to the choice of electrode materials. Graphene offers advantage of transparency, flexibility and potential low cost. The process of self-limiting nanogap generation in the graphene layer in the planar G-SiO x -G memory system is an advantage of graphene that otherwise may not be assumed by other transparent materials. Given the unique role of SiO x in the semiconductor industry and the promising future of graphene as a transparent electrode material, the SiO x –graphene memory system demonstrated here features its advantages in both transparent materials composition and processing. Material preparation The graphene films were synthesized directly on 25 μm thick copper foils (Alfa Aesar, 99.8%) via the chemical vapour deposition method [24] . The process began with the thermal annealing of the copper foil at 1,035 °C under H 2 flow (500 sccm) for 20 min for grain coarsening. Then at the stabilized temperature of 1,035 °C and pressure of 10 Torr, CH 4 precursor gas (4 sccm) was introduced into the growth tube for graphene growth (40 min). After that, the CH 4 flow was turned off and the furnace was cooled down to room temperature. Protected with poly(methyl methacrylate), the graphene-coated copper film was then etched in a Fe(NO 3 ) 3 solution (0.5 M), followed by thoroughly cleaning in a 5% HNO 3 solution and deionized (DI) water. Fabrication of G/SiO x /ITO pillar structure The schematic of the fabrication is presented in Supplementary Fig. S1 . A glass substrate coated with an ITO layer (120 nm, ~100 Ω sq −1 ) was used as the starting substrate. A layer of SiO x (~70 nm thick) was deposited by electron-beam evaporation. Then monolayer graphene film was transferred (twice for bilayer) on to the SiO x /ITO/glass substrate to form the graphene top electrode. For the definition of the circular patterns, photolithography was used to define circular resist (Microposit S1813) patterns (diameters ~100 μm) as the sacrificial mask. Reactive ion etching (RIE, using CHF 3 /O 2 ) was then used to vertically etch the graphene and SiO x layer at the region unprotected by the resist. The resist mask was then removed by acetone. Note that an etched vertical SiO x (red arrow, Supplementary Fig. S1 ) is necessary for the electroforming process and the subsequent memory switching, as the etched surface is expected to be more defected compared with the rest bulk region in the SiO x layer and, hence, provides the localized region for the self-limiting process of silicon filament formation [17] . Fabrication of G/SiO x /G pillar structure The schematic of the fabrication is presented in Supplementary Fig. S5 . To form the layered structure of G/SiO x /G, a bilayer graphene film (using layer-by-layer transferred technique) was first transferred onto the glass substrate. A layer of SiO x film with the thickness of 70 nm was deposited by electron-beam evaporation. The top bilayer graphene film was then transferred on to the SiO x layer. Circular resist patterns (diameters ~100 μm) were then defined by photolithography as described above. Oxygen plasma was used to etch the top graphene film at the region unprotected by the resist mask. RIE (CHF 3 /O 2 ) was then used to partially etch the SiO x layer followed by further SiO x etching by buffered oxide etch (10:1). The reason for adopting the two-step SiO x etching is to protect the bottom graphene electrodes from RIE etching while still define the vertical SiO x edge that facilitates the electroforming [17] . The resist was then removed with acetone. The fabrication of G/SiO x /G pillar structures on the plastic substrate followed the similar procedure. In addition, the fluoropolymer (operational temperature larger than 280 °C; purchased from McMaster) plastic substrate was treated with oxygen plasma for 90 s to increase its wettability to acetone, before the transfer of the bottom bilayer graphene films. After the oxygen plasma treatment, the measured contact angle with acetone decreases from 69.3° to 25.7°. For easier handling of the plastic substrate, it was fixed on a silicon substrate during the fabrication process. Fabrication of G/SiO x /G crossbar structure The G/SiO x /G crossbar structure was fabricated on a silicon substrate ( ρ >5,000 Ω cm) and plastic substrate (fluoropolymer). The bottom bilayer graphene was first transferred on to the silicon substrate or plastic substrates. Transferring bottom graphene to plastic substrates follows the same procedure for the fabrication of G/SiO x /G pillar structures on fluoropolymer. Photolithography was used to define the resist mask, and then oxygen plasma was used to etch and define the bottom graphene lines as shown in Fig. 3a . Metal electrode (Au/Ti=20 nm/2 nm, 100×100 μm 2 ) was patterned at the end of each graphene line by photolithography, electron-beam evaporation and lift-off processes, serving as the bottom electrical contact for the probe tip. A layer of SiO x film (~70 nm) was then deposited by electron-beam evaporation. The top bilayer graphene film was then transferred onto the SiO x layer. Photolithography was used to define the sacrificial layer for the top graphene lines, followed by the two-step SiO x etching method described before. Finally, top-metal electrode (Au/Ti=30 nm/5 nm, 100×100 μm 2 ) was also patterned at the end of each top graphene line to form electrical contact for the upper probe tip. How to cite this article: Yao, J. et al . Highly transparent nonvolatile resistive memory devices from silicon oxide and graphene. Nat. Commun. 3:1101 doi: 10.1038/ncomms2110 (2012).